The oldest North American pachycephalosaurid and the hidden diversity of small-bodied ornithischian dinosaurs Taphonomic biases dictate how organisms are represented in the fossil record, but their effect on studies of vertebrate diversity dynamics is poorly studied. In contrast to the high diversity and abundance of small-bodied animals in extant ecosystems, small-bodied dinosaurs are less common than their large-bodied counterparts, but it is unclear whether this reflects unique properties of dinosaurian ecosystems or relates to taphonomic biases. A new, fully domed pachycephalosaurid dinosaur, Acrotholus audeti , from the Santonian of Alberta predates incompletely domed taxa, and provides important new information on pachycephalosaur evolution and the completeness of the ornithischian fossil record. Here we provide the first empirical evidence that the diversity of small-bodied ornithischian dinosaurs is strongly underestimated based on ghost lineages and the high proportion of robust and diagnostic frontoparietal domes compared with other pachycephalosaur fossils. This suggests preservational biases have a confounding role in attempts to decipher vertebrate palaeoecology and diversity dynamics through the Mesozoic. The diversity dynamics of dinosaurs through the Mesozoic era and their pattern of species richness leading up to the end Cretaceous extinction event continue to be hotly debated [1] , [2] , [3] , [4] , [5] . Recent studies have emphasized the influence of sampling biases on our understanding of vertebrate diversity patterns through time, but have focused on identifying and correcting for uneven sampling intensity [2] , [6] , [7] . Taphonomic biases in the form of selective preservation dictate how organisms are preserved and enter the fossil record, but the effect of these biases on large-scale palaeontological studies of vertebrate diversity dynamics and quantitative macroevolutionary patterns have been comparatively poorly studied [8] . The bones of large-bodied terrestrial vertebrates are often better represented in fossil assemblages than their small-bodied counterparts because of strong taphonomic biases against the preservation of small vertebrates in a variety of host systems [8] , [9] , [10] . These factors have significant potential to effect perceptions of diversity dynamics of vertebrates through time. In contrast to the comparatively high diversity and abundance of small-bodied mammals and reptiles in extant ecosystems [11] , [12] , small-bodied (<100 kg) dinosaurs are considerably less common than their large-bodied counterparts in most well-sampled assemblages throughout the Mesozoic [13] . This paradox is further underscored by the apparent rarity of small, herbivorous ornithischians when compared with the diversity of small-bodied theropods [13] , [14] . Furthermore, it has been suggested that ontogenetic niche shifts within large-bodied dinosaur taxa are responsible for the perceived low α-diversity of small- and medium-sized dinosaurs (1–1,000 kg) [15] . Whether this pattern reflects a unique property of dinosaurian ecosystems or is an artifact of taphonomic or other biases has not been addressed, but species fidelity in dinosaur fossil assemblages could have major implications for studies of dinosaur palaeocology and diversity dynamics over both large and small timescales. Pachycephalosaurs (Ornithischia: Marginocephalia) are an enigmatic group of primarily small-bodied herbivorous ornithischians characterized by thickened cranial domes [16] , [17] that are integral to understanding patterns of ornithischian evolution, as well as the function and evolution of bizarre structures in dinosaurs [18] , [19] , [20] , [21] . Here we describe fossils of a new pachycephalosaur from Santonian-aged deposits of Alberta, Canada, which represent the oldest unequivocal member of this clade from North America [16] , [19] , [21] , [22] , and possibly the world [23] . This new taxon predates all putatively more primitive and incompletely domed taxa, yet is remarkable for having a fully developed cranial dome, and therefore provides additional information on the evolutionary timing of their distinctive cranial characters and the completeness of the pachycephalosaur fossil record. The special taphonomic properties of pachycephalosaurs’ robust cranial domes, including frequent preservation and phylogenetically informative morphology that is diagnostic to low taxonomic levels, provide a unique opportunity to address the nature of the small-bodied dinosaur fossil record, with implications for studies of palaeoecology and diversity dynamics. Systematic palaeontology. Dinosauria Owen 1842 Ornithischia Seeley 1888 Pachycephalosauridae Sternberg 1945 Acrotholus audeti gen. et. sp. nov. Etymology. From the Greek akros , meaning highest, and tholos , meaning dome; in reference to its greatly thickened cranial vault. The specific epithet honours Roy Audet, for allowing access to his ranch where the holotype skull was found. Type series. TMP (Royal Tyrrell Museum of Palaeontology) 2008.045.0001 (holotype), nearly complete frontoparietal dome ( Fig. 1 ; Supplementary Fig. S1 ; DigiMorph); ROM (Royal Ontario Museum) 2962 (paratype), anterior half of frontoparietal dome ( Fig. 2 ). Locality and horizon. TMP 2008.045.0001, ROM 2962 and ROM 2964 ( Supplementary Fig. S2 ) were collected from the Deadhorse Coulee Member of the Milk River Formation exposed in southern Alberta, Canada (see Supplementary Note S1 and Supplementary Figs S3 and S4 ). The holotype was recovered 1.5 km east of Writing-On-Stone Provincial Park, 22.9 m above the base of the Deadhorse Coulee Member. ROM 2962 and ROM 2964 have less precise stratigraphic data, but both specimens were collected ∼ 9.5 km east of Writing-On-Stone Provincial Park in exposures adjacent to Black Coulee (formerly Deadhorse Coulee). The Deadhorse Coulee Member of the Milk River Formation has been dated as Late Santonian in age (see Supplementary Note S1 ). Detailed locality data is on file at the TMP and ROM. Diagnosis. Medium-sized pachycephalosaurid with the following autapomorphies: ovoid dome in dorsal view in which the width of the frontoparietal dome is less than two thirds its total length, distinct midline ridge on the dorsal surface of the posteromedian process of the parietal. Differs from Stegoceras validum and Colepiocephale in the absence of grooves between the frontonasal boss and the supraorbital lobe, the full incorporation of supraorbitals into the dome, and in the symmetry of the dome in lateral view. Differs from Pachycephalosaurus and Sphaerotholus in that the postorbital extends higher on the dome than the posterior supraorbital, and their sutural surfaces are strongly arched dorsally. Comments. Sullivan [16] , [24] described ROM 2964, an incomplete, poorly preserved dome from the Milk River Formation, showing clear signs of pathology, but was not able to assign it to a particular taxon or assess its phylogenetic position. ROM 2964 has a similar overall shape to TMP 2008.045.0001, and may be referable to the new taxon ( Supplementary Fig. S2 ). 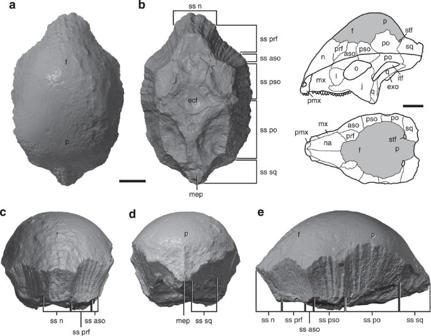Figure 1: Holotype specimen ofAcrotholus audeti. Surface scan image captures of TMP 2008.045.0001 in (a) dorsal, (b) ventral, (c) anterior, (d) posterior and (e) left lateral views. aso, anterior supraorbital; exo, exoccipital; f, frontal; itf, infratemporal fenestra; j, jugal; l, lacrimal; mep, median extension of the parietal; mx, maxilla; n, nasal; o, orbit; p, parietal; pmx, premaxilla; po, postorbital; prf, prefrontal; pso, posterior supraorbital; q, quadrate; qj, quadratojugal; sq, squamosal; ss aso, sutural surface for the anterior supraorbital; ss n, sutural surface for the nasal; ss po, sutural surface for the postorbital; ss prf, sutural surface for the prefrontal; ss pso, sutural surface for the posterior supraorbital; ss sq, sutural surface for the squamosal; stf, supratemporal fenestra. Scale bar equals 2 cm ina–e, and 5 cm for the inset skull diagram. Figure 1: Holotype specimen of Acrotholus audeti . Surface scan image captures of TMP 2008.045.0001 in ( a ) dorsal, ( b ) ventral, ( c ) anterior, ( d ) posterior and ( e ) left lateral views. aso, anterior supraorbital; exo, exoccipital; f, frontal; itf, infratemporal fenestra; j, jugal; l, lacrimal; mep, median extension of the parietal; mx, maxilla; n, nasal; o, orbit; p, parietal; pmx, premaxilla; po, postorbital; prf, prefrontal; pso, posterior supraorbital; q, quadrate; qj, quadratojugal; sq, squamosal; ss aso, sutural surface for the anterior supraorbital; ss n, sutural surface for the nasal; ss po, sutural surface for the postorbital; ss prf, sutural surface for the prefrontal; ss pso, sutural surface for the posterior supraorbital; ss sq, sutural surface for the squamosal; stf, supratemporal fenestra. Scale bar equals 2 cm in a – e , and 5 cm for the inset skull diagram. 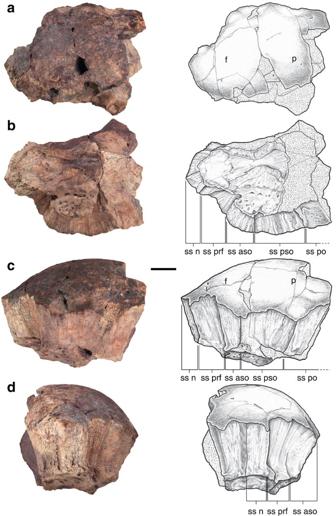Figure 2: Paratype specimen ofA. audetiwith interpretive drawings. (a) Dorsal, (b) ventral, (c) left lateral and (d) anterior views. Abbreviations as inFig. 1. Scale bar, 2 cm. Full size image Figure 2: Paratype specimen of A. audeti with interpretive drawings. ( a ) Dorsal, ( b ) ventral, ( c ) left lateral and ( d ) anterior views. Abbreviations as in Fig. 1 . Scale bar, 2 cm. Full size image Comparative description The new frontoparietal material includes a complete, well-preserved frontoparietal ( Fig. 1 and Supplementary Fig. S1 ), and a second, equally well-preserved specimen that consists of the frontal region of the cranial dome ( Fig. 2 ). The elongate ovoid shape of the dome in A. audeti is distinct from all known pachycephalosaurid taxa. The thickened domes are relatively large and notably massive, with a maximum thickness above the cerebral fossa (55 mm) of almost half of the total length in TMP 2008.015.0001. The apex of the frontoparietal dome occurs centrally, such that it is symmetrical in lateral view, with a slight depression over the parietal region. The dorsal dome surface is devoid of tesserae or minute tubercles that are characteristic of ‘flat-headed’ pachycephalosaurs and juveniles of domed taxa, which is probably indicative of a relatively mature ontogenetic stage for the known specimens [25] , [26] , [27] , [28] . Histological data from high-resolution computed tomography (CT) scans show extremely low relative vascularity, high density and fully internally fused frontal–frontal and frontoparietal sutures in the holotype specimen ( Fig. 3 ), which further supports a mature ontogenetic stage for this specimen (see Supplementary Methods ). The dorsally convex frontonasal boss is short relative to Stegoceras validum (e.g., University of Alberta Laboratory for Vertebrate Paleontology 2 and Colepiocephale lambei ), and it is not separated from the anterior supraorbital lobe by grooves that characterize Campanian-aged pachycephalosaurid taxa from North America [25] . The dorsoventral thickness of the boss is ∼ 50% that of the thickest region of the dome (55 mm) above the cerebral fossa. 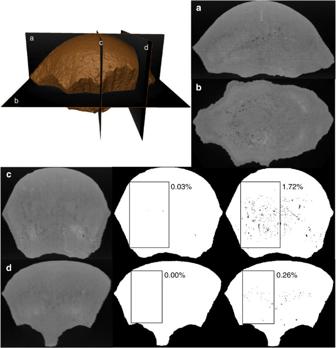Figure 3: High-resolution computed tomography scans of the holotype specimen ofA. audeti. Top left, a three-dimensional model built from the CT scans and the various planes that were digitally sectioned; top right and bottom left, CT scans in various orientations; bottom middle and right, thresholded images, with region of interest and void space calculation shown using the Huang method (middle) and manual thresholding (right). (a) Sagittal section; (b) frontal section; (c) transverse section at the junction of the posterior supraorbital and postorbital sutures; (d) transverse section at the frontoparietal suture. Note the low-void (vascular) space, the high density (light colour) and the lack of frontal–frontal or frontoparietal sutures. Figure 3: High-resolution computed tomography scans of the holotype specimen of A. audeti . Top left, a three-dimensional model built from the CT scans and the various planes that were digitally sectioned; top right and bottom left, CT scans in various orientations; bottom middle and right, thresholded images, with region of interest and void space calculation shown using the Huang method (middle) and manual thresholding (right). ( a ) Sagittal section; ( b ) frontal section; ( c ) transverse section at the junction of the posterior supraorbital and postorbital sutures; ( d ) transverse section at the frontoparietal suture. Note the low-void (vascular) space, the high density (light colour) and the lack of frontal–frontal or frontoparietal sutures. Full size image The position, morphology and relative size of the vertically striated sutural surfaces for the peripheral elements are nearly identical in TMP 2008.015.0001 and ROM 2962, where preserved in both specimens. The sutural surfaces for the peripheral bones are very well developed and high on the dome, indicating that the peripheral bones were completely incorporated into the dome. The posterior supraorbital sutural surface and the combined prefrontal–anterior supraorbital sutural surface are subequal in size, approximately half that of the massive sutural surface for the postorbital. The anterior supraorbital sutural surface is limited to only a thin-slip anterior to the sutural surface for the posterior supraorbital. The extent that the supraorbitals are incorporated into the dome is equal to, or surpasses, that in ‘fully domed’ pachycephalosaurids, such as Pachycephalosaurus and Prenocephale , and is notably greater than in Stegoceras validum and Colepiocephale lambei . The dorsal margins of the posterior supraorbital and the postorbital sutural surfaces are strongly arched, resulting in a small diastema between these bones, as in Stegoceras and Prenocephale , but unlike Sphaerotholous and Pachycephalosaurus . The rugose region posterior to the postorbital sutural surface represents the sutural surface for the squamosal. The cranial roof exceeds 15 mm in thickness over the supratemporal fossa, and it is clear that supratemporal fenestrations are absent (that is, the supratemporal fenestrae are closed). In dorsal view, the posteromedian extension of the parietal tapers posteriorly to a blunt point. Its dorsal surface bears a raised midline ridge that extends to the distal end of the parietal. A ridge of fused nodes occurs on some juvenile specimens of Stegoceras validum (for example, University of Calgary Museum of Zoology 2008.01), but these are never raised above the rest of the parietal surface, particularly in large specimens (UALVP 2). This posterior end of the posteromedian process is slightly damaged in the holotype. However, the sutural surface for the left squamosal extends to the posterior end of the posteromedian process, such that the squamosals could have only been separated by a very thin slip of the parietal, if at all, along the posterior margin of the parietosquamosal bar. Hypertrophied nodes indicative of a parietosquamosal node row are absent on the parietal. The dorsal surface of the parietal is slightly depressed above of the posterior region of the temporal chambers, as in Sphaerotholus goodwini and Prenocephale prenes , but it lacks a stepped transition to a prominent parietosquamosal shelf, as in Colepiocephale lambei [29] and variably present in Stegoceras validum [24] , [30] . The lateral profile of the parietal suggests a weakly developed parietosquamosal shelf intermediate in morphology between the horizontal posteromedian extension of the parietal of Stegoceras validum and the smoothly rounded parietal morphology (sometimes referred to as ‘down-turned’) of Sphaerotholus and Prenocephale [24] , [25] . The ventral surface of the frontoparietal dome has three major depressions: the orbital cavity, the endocranial fossa and the temporal fossa. The total length of the endocranial fossa in the holotype measures 35 mm from the anterior end of the olfactory bulbs to the posterior margin of the cerebral fossa, and the maximum width of the bulbs is ∼ 40% that of the widest point of the endocranial cavity (25 mm). The large olfactory bulbs join the anterior end of the cerebral fossa via short olfactory peduncles, as is typical in pachycephalosaurids. The distinctly rugose sutural surface for the attachment of the sphenoid bones separates the orbital cavity from the endocranial fossa. The orbital fossae are only slightly concave and pierced by a large number of small foramina. Posterior to the cerebral fossa, the parietal is broken above the level of contact with the supraoccipital. Here it forms a thick midline bridge that extends from the endocranial fossa to the posterior end of the skull and separates the left and right temporal fossae. The roof of the temporal chamber is weakly arched, with a rugose scarring for temporal muscle attachment medially, and a relatively smooth lateral surface pierced by a series of small foramina. In lateral view, the roof of the temporal chamber is shallowly inclined, but not highly arched as in Sphaerotholus [25] . Morphometric analyses Allometric analyses ( Fig. 4a , Table 1 , see also Supplementary Methods , Supplementary Figs S5–S7 and Supplementary Table S1 ) show that numerous aspects of cranial form are strongly related to size in the sample, with poor taxonomic distinction. The thickness of the dome and the height of the nasal boss are positively allometric contrary to Chapman et al. [31] and do not show significant differences among the taxa in the sample. Variability is greatest in the degree to which the supraorbital bones are incorporated into the dome (H:aso/pso). Stegoceras validum differs from other taxa in having lower supraorbital joint surfaces, especially compared with those in Prenocephale -grade taxa. A. audeti is notable for the massively thickened supraorbital region of the skull, and the full incorporation of the supraorbitals into the dome ( Fig. 4 ). 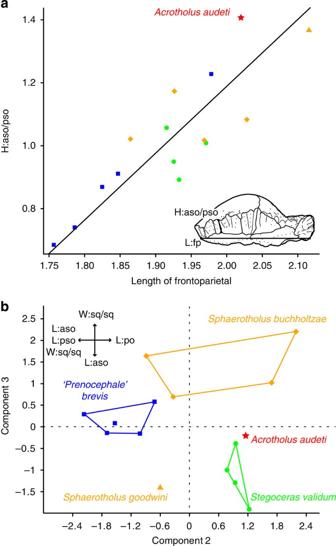Figure 4: Selected results of morphometric analyses of pachycephalosaur frontoparietal domes. (a) Plot of supraorbital height against frontoparietal length, with RMA regression line, illustrating the distinct nature ofA. audetiin this feature. (b) Plot of second and third PCs of the PCA (which were not correlated with size, seeSupplementary Note S2) illustrating thatAcrotholusfalls outside the morphospace occupied by the other taxa. Star,A. audeti; circle,Stegoceras validum; square,Prenocephale brevis; diamond,Sphaerotholus buchholtzae; triangle,Sphaerotholus goodwini. Measurements inaare log-transformed (mm). The inset in the upper left ofbdepicts the measurements, which load most strongly in each direction. Outlines inbare convex hulls around taxa. H:aso/pso, height of the sutural surface at the contact of the anterior supraorbital and posterior supraorbital; W:sq/sq, width between the squamosal suture just ventral to the node row. L:aso, length of the anterior supraorbital suture; L:pso, length of the posterior supraorbital suture; L:po, length of the postorbital suture; L:fp, length of the frontoparietal. Figure 4: Selected results of morphometric analyses of pachycephalosaur frontoparietal domes. ( a ) Plot of supraorbital height against frontoparietal length, with RMA regression line, illustrating the distinct nature of A. audeti in this feature. ( b ) Plot of second and third PCs of the PCA (which were not correlated with size, see Supplementary Note S2 ) illustrating that Acrotholus falls outside the morphospace occupied by the other taxa. Star, A. audeti ; circle, Stegoceras validum ; square, Prenocephale brevis ; diamond, Sphaerotholus buchholtzae ; triangle, Sphaerotholus goodwini . Measurements in a are log-transformed (mm). The inset in the upper left of b depicts the measurements, which load most strongly in each direction. Outlines in b are convex hulls around taxa. H:aso/pso, height of the sutural surface at the contact of the anterior supraorbital and posterior supraorbital; W:sq/sq, width between the squamosal suture just ventral to the node row. L:aso, length of the anterior supraorbital suture; L:pso, length of the posterior supraorbital suture; L:po, length of the postorbital suture; L:fp, length of the frontoparietal. Full size image Table 1 Results of bivariate allometric analyses of Pachycephalosaur frontoparietal dimensions. Full size table A principle component analysis (PCA) was conducted on the data set using the software program PAST [32] for the correlation matrix. The oblong dome of A. audeti is separated from all other taxa in the PC morphospace, supporting its recognition as a distinct taxon ( Fig. 4b ). The first three principal components (PCs) account for 93% of the total variation in the data set (see Supplementary Tables S2 and S3 ). PC1 accounts for the majority of the total variance in the sample (71%). It is strongly correlated with frontoparietal length ( r =0.93) and most other variables (except W:sq/sq and to a lesser extent L:aso) load strongly, and in the same direction, onto this component, indicating it is largely related to size. PC2 and PC3 do not show significant correlations with frontoparietal length ( r =−0.14 and 0.13, respectively), and so reflect variation that may be most phylogenetically informative. Four variables show loadings with magnitudes greater than 0.3 on PC2: L:aso, L:pso, W:sq/sq loaded negatively and L:po loaded positively. Two variables are strongly associated with PC3: W:sq/sq (positive) and L:aso (negative). The plot of PC2 versus PC3 ( Fig. 4b ) shows that Prenocephale -grade taxa are relatively tightly clustered together, whereas specimens of Stegoceras validum, including Ornatotholus browni [28] , at several stages of development are more widely dispersed, but do not overlap with Prenocephale -grade taxa. Phylogenetic analysis A phylogenetic analysis of 16 pachycephalosaurian in-group taxa and 50 morphological characters resulted in 13 most parsimonious trees ( Supplementary Methods , Supplementary Note S2 , Supplementary Table S4 and Supplementary Fig. S8 ). A time-calibrated phylogeny of the most stratigraphically consistent MPT is shown in Fig. 5 . The time calibration reveals substantial missing diversity in the pachycephalosaur fossil record, which would be considerably greater without taxa known only from their robust domes ( Fig. 5 ). 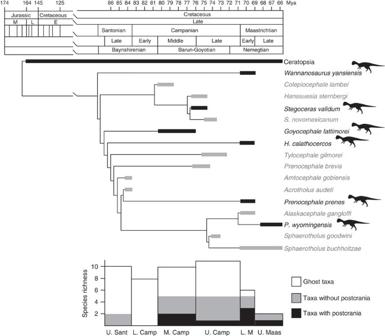Figure 5: Time-calibrated phylogenetic tree of Pachycephalosauria. Parsimony analysis resulted in 13 most parsimonious trees, with a Tree Length of 68 steps, a Consistency Index of 0.72 and a rescaled Consistency Index of 0.58. The most stratigraphically consistent tree (also the tree with the best Gap Excess Ratio, seeSupplementary Methods) was used for time calibration. Time-calibrated results indicate substantial missing diversity in the pachycephalosaur fossil record, which would be considerably greater without taxa known only from their taphonomically robust domes. Taxa indicated with grey are known only from cranial material, and those in black are known from postcranial remains. Bar graph (bottom) tracks species richness of pachycephalosaurs, taxa with postcrania (black), taxa known from isolated cranial material only (grey) and inferred based on ghost lineages from the phylogeny (white). Figure 5: Time-calibrated phylogenetic tree of Pachycephalosauria. Parsimony analysis resulted in 13 most parsimonious trees, with a Tree Length of 68 steps, a Consistency Index of 0.72 and a rescaled Consistency Index of 0.58. The most stratigraphically consistent tree (also the tree with the best Gap Excess Ratio, see Supplementary Methods ) was used for time calibration. Time-calibrated results indicate substantial missing diversity in the pachycephalosaur fossil record, which would be considerably greater without taxa known only from their taphonomically robust domes. Taxa indicated with grey are known only from cranial material, and those in black are known from postcranial remains. Bar graph (bottom) tracks species richness of pachycephalosaurs, taxa with postcrania (black), taxa known from isolated cranial material only (grey) and inferred based on ghost lineages from the phylogeny (white). Full size image Pachycephalosaur taphonomy Analysis of preservational modes using a global database of virtually all known non-dental pachycephalosaur specimens ( n =575) illustrates that the vast majority of specimens consist of isolated cranial elements (86%) with comparatively few isolated postcranial elements, and even fewer associated or articulated skeletons ( Fig. 6a , see also Supplementary Table S5 ). This pattern is consistent across all North American collections and formations, with the isolated cranial dome material always making up more than three quarters of the specimens, and often making up a much greater proportion. This indicates that the pattern of preservation is not driven by properties of individual formations or historical collecting practices, but is a consistent pattern for the North American pachycephalosaur fossil record. Available data from Asia suggests that this pattern may not be as strong in representative Asian formations, but the sample sizes are exceedingly small and with fewer independent samples. 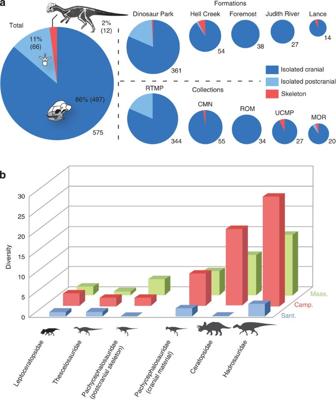Figure 6: Preservational modes in Pachycephalosauria and comparative diversity of Ornithischians. (a) Relative taphonomic representation of global Pachycephalosauria specimens (Supplementary Table S6). Pie chart on left indicates total sample, charts on top are segregated by formation and those on the bottom are segregated by collection. Dark blue indicates cranial specimens (specifically the thickened cranial dome and peripheral elements), light blue indicates isolated postcranial elements and red indicates articulated or associated skeletons. In all cases, sample size (lower right of each circle) decreases to the right and the size of the circle is scaled relative to the sample size. (b) Global diversity (number of species) of major Late Cretaceous ornithischian clades in the Santonian (blue), Campanian (red) and Maastrichtian (green) (Supplementary Table S7). Clades comprising small-bodied taxa are on the left (Leptoceratopsidae and Thescelosauridae), show a similar, low diversity compared with clades comprised predominantly of large taxa on the right (Hadrosauridae and Ceratopsidae). When tallied on the basis of taxa known from any postcranial material, pachycephalosaurs exhibit low diversity comparable to that of other small-bodied groups (center left). The relatively high diversity of pachycephalosaurs compared with other contemporaneous small-bodied dinosaur groups is driven by isolated cranial dome elements (centre right). Figure 6: Preservational modes in Pachycephalosauria and comparative diversity of Ornithischians. ( a ) Relative taphonomic representation of global Pachycephalosauria specimens ( Supplementary Table S6 ). Pie chart on left indicates total sample, charts on top are segregated by formation and those on the bottom are segregated by collection. Dark blue indicates cranial specimens (specifically the thickened cranial dome and peripheral elements), light blue indicates isolated postcranial elements and red indicates articulated or associated skeletons. In all cases, sample size (lower right of each circle) decreases to the right and the size of the circle is scaled relative to the sample size. ( b ) Global diversity (number of species) of major Late Cretaceous ornithischian clades in the Santonian (blue), Campanian (red) and Maastrichtian (green) ( Supplementary Table S7 ). Clades comprising small-bodied taxa are on the left (Leptoceratopsidae and Thescelosauridae), show a similar, low diversity compared with clades comprised predominantly of large taxa on the right (Hadrosauridae and Ceratopsidae). When tallied on the basis of taxa known from any postcranial material, pachycephalosaurs exhibit low diversity comparable to that of other small-bodied groups (center left). The relatively high diversity of pachycephalosaurs compared with other contemporaneous small-bodied dinosaur groups is driven by isolated cranial dome elements (centre right). Full size image Ornithischian diversity Records of ornithischian α-diversity through the final three stages of the Cretaceous, obtained from the Paleobiology Database ( http://paleodb.org/ ), were compiled and compared ( Supplementary Table S6 ). The results show that clades comprised predominantly of small-bodied taxa (Leptoceratopsidae, Thescelosauridae) exhibit low diversity compared with those clades dominated by large-bodied taxa (Hadrosauridae, Ceratopsidae). Pachycephalosaur diversity is much higher than clades that exhibit a similar body size range, especially in the Campanian and Maastrichtian, but this is only true when a large number of taxa represented only by frontoparietal domes are included. Otherwise, the diversity of pachycephalosaurs compares readily with the other small-bodied ornithischian groups ( Fig. 6b ). A new phylogenetic analysis recovers A. audeti as the sister taxon to Prenocephale prenes from the Maastrichtian of Mongolia ( Fig. 5 ). The flat-headed Wanannosaurus is recovered as the sister taxon to all other pachycephalosaurs, consistent with most previous analyses [17] , [24] , [25] , [30] . However, Goyocephale and Homalocephale are more closely related to fully domed taxa, including A. audeti , P. prenes and pachycephalosaurines, than they are to Stegoceras , and are not outside the clade of domed pachycephalosaurs as is traditionally thought [30] . This supports the recent hypothesis that these taxa may represent juvenile individuals of domed taxa [27] , [28] , [33] . Recent reviews have questioned the taxonomic assignment of the putative earliest members of the clade, including Yaverlandia, Stenopelix and Ferganocephale , and concluded that there is no clear evidence of pachycephalosaurs before the Santonian [16] , [22] . As a result, the early evolutionary history of the group is one of the most poorly understood aspects of dinosaurian evolution [16] , [19] , [22] , [34] . The Late Santonian age of A. audeti predates all other pachycephalosaurs from North America [16] , [24] . Other reports of older pachycephalosaurs based on isolated teeth are unsubstantiated [16] , [35] , [36] . Other skull material appears in the North American fossil record in the middle Campanian [16] , [28] , approximately five million years after Acrotholus . Acrotholus also predates the well-known series of Asian pachycephalosaurs, including the flat-headed taxa Goyocephale and Homalocephale [16] , [37] . Watabe et al. [23] recently described the oldest unequivocal pachycephalosaur from Asia based on a frontoparietal from the upper Bayn Shireh Formation of Mongolia, which has been suggested to be Santonian in age [38] , approximately equivalent in age to Acrotholus . The thickened and highly vaulted dome in A. audeti demonstrates that numerous traits associated with derived pachycephalosaurs (completely closed supratemporal fenestrae, loss of a prominent posterior parietosquamosal shelf, complete incorporation of the supraorbital bones into the dome) evolved at least by the Santonian stage of the late Cretaceous and well before the first appearance of putatively flat-headed ( Goyocephale , Homalocephale and Wannanosaurus ) and incompletely domed taxa (for example, Stegoceras validum , Colepiocephale lambei ) that are often hypothesized to exhibit primitive pachycephalosaur traits [17] , [24] , [25] , [30] . Temporal calibration of the phylogenetic tree suggests major sampling issues in the fossil record of Pachycephalosauria ( Fig. 5 ). Although this approach is sensitive to phylogenetic accuracy [39] , [40] , ghost lineages calculated from the phylogeny suggest that the diversity of pachycephalosaurs is severely underestimated, perhaps by a factor of five times or more in well-sampled intervals of the middle and late Campanian [2] . This poor sampling is corroborated by the strongly supported sister group relationship between Pachycephalosauria and Ceratopsia [18] , [21] , which results in a massive ghost lineage that spans from the late Jurassic (Oxfordian) occurrence of Yinlong downsi , the earliest known ceratopsian, to A. audeti , a span of at least 66 million years that encompasses globally well-sampled intervals in the latest Jurassic and early Cretaceous [2] . The small size of most pachycephalosaurs [41] , typically less than 40 kg, makes them among the smallest ornithischian dinosaur taxa. Actualistic taphonomic experiments that demonstrate strong biases against the preservation of small-bodied terrestrial vertebrates in a variety of host systems [8] , [9] suggest that the diversity of small-bodied dinosaur taxa may be dramatically underestimated in the fossil record. Taphonomic biases against preservation of small species appears to be due to the greater susceptibility of small bones to destruction by carnivores, breakage through bioturbation and weathering processes [8] , [9] , [42] . Unlike their relatively delicate postcranial remains, the massively constructed frontoparietal domes of pachycephalosaurids are robust elements resistant to predepositional destruction. They are also phylogenetically informative, diagnostic to the species level and are easy to recognize in the field. Not surprisingly, the robust frontoparietal domes and associated peripheral elements account for the vast proportion of the pachycephalosaur fossil record ( Fig. 6a ). Isolated cranial remains of pachycephalosaurs in museum collections (for example, the American Museum of Natural History, the Canadian Museum of Nature, ROM and TMP) outnumber postcranial remains by a factor of at least 7 to 1 ( Fig. 6a ). In terms of skeletal representation of individual taxa, greater than 66% of named taxa are known strictly from cranial material (predominantly frontoparietal domes), and only six taxa have any associated postcrania. As such, the ratio of observed to true diversity is likely to be higher for pachycephalosaurs than for other similar small-bodied ornithischians that lack such robust, diagnostic skeletal elements. When only taxa with known postcrania are considered, the pachycephalosaur fossil record closely resembles those of other small-bodied ornithischians, where there are relatively few taxa with reasonably complete skeletons that are widely distributed in time and space (such as heterodontosaurs [43] , [44] , thescelosaurids and other small-bodied ornithopods [45] , [46] , and leptoceratopsids [47] ; Fig. 6b ). In modern terrestrial mammal dominated faunas, field surveys conducted by Behrensmeyer et al. [9] noted that all mammal species greater than 100 kg body mass were easily recognized in their sampled bone assemblages, but that species fidelity of smaller species in the same bone assemblages was inversely related to body size. Terrestrial vertebrate fossil assemblages of Mesozoic age are typically derived from alluvial deposits that preserve evidence for bone or carcass transport and reworking [48] , [50] . In these deposits, small skeletons are rare relative to those of large dinosaurs [42] , [49] , [50] . Unlike mammals, the less complex and stereotyped tooth morphology in most major dinosaur groups provides poor information on α-diversity patterns at low taxonomic levels, and therefore microvertebrate assemblages likely provide little meaningful insights into the species richness of small-bodied dinosaurs. Extensive work on variation in small theropod teeth over the last three decades has allowed modest resolution of their diversity in vertebrate microfossil assemblages [51] , [52] , [53] , but the generalized foliform morphology of isolated ornithischian teeth has made inferences of taxonomic diversity in small-bodied herbivorous dinosaurs based on vertebrate microfossil assemblages much more difficult [2] , [54] , beyond the presence or absence of major groups [22] , [55] . Pachycephalosaurs likely had broadly similar ecological requirements and, with the exception of the robust frontoparietal domes, had comparable preservation potential to other groups of small-bodied ornithischian dinosaurs, including leptoceratopsids, small-bodied ornithopods and heterodontosaurs. If estimates of missing diversity implied by the unique fossil record of pachycephalosaurs can be extended to these other small-bodied ornithischian groups, their true α-level diversity is also extremely poorly known. The same is likely true for small theropods [49] . The unique nature of the pachycephalosaur record provides empirical evidence that α-level diversity of small-bodied ornithischian dinosaurs is strongly underestimated. The scant fossil record of small-bodied dinosaurs in general [56] , [57] , [58] , [59] indicates preservational biases have a major, confounding role in attempts to model the diversity dynamics and ecology of dinosaur-dominated ecosystems through the Mesozoic Era. Relatively high recovery potential of small-bodied dinosaur diversity is likely tied to lagerstätten, which are non-randomly distributed in time and space [60] . Because of this, overall patterns of small-bodied dinosaur diversity are heavily influenced by lagerstätten effects, which confound methods attempting to control for sampling intensity, particularly model-based approaches generated using regression methods [1] , [2] , [6] , [7] . Future studies of diversity dynamics should attempt to control for these body size biases in species fidelity, perhaps by focusing on large-bodied taxa given their higher probability of preservation and recovery in alluvial and other continental depositional settings [9] , as well as analysing taphonomically equivalent depositional settings. Frontoparietal bone histology High-resolution CT scans of the holotype specimen of A. audeti , TMP 2008.045.0001, were performed to examine the gross histology of this specimen and calculate its relative void space, a proxy for vascularity [28] . See Supplementary Methods for additional details. Morphometric analyses To assess the range of variation in the shape of pachycephalosaurid domes and test the morphological distinctiveness of A. audeti , we measured 15 landmark-based indices based on those of Schott et al. [28] on 15 complete, non-pathological pachycephalosaurid domes from five small-bodied taxa from the late Cretaceous of North America ( Supplementary Table S1 ). Using these measurements, we conducted a series of bivariate analyses and a PCA to test the distinctiveness of Acrotholus , and assess size and shape variation in pachycephalosaurs. All measurements were log-transformed to fit the linear allometric growth function before analysis, and total length of the frontoparietal (L:fp) was used as the standard ( x ) variable for the bivariate plots. This measurement was not included in the PCA, to allow us to test for size dependence of the PCs. PCA results in Fig. 4b were obtained using the correlation matrix (although both were tested), which gives equal weight to measurements of varying magnitude. See Supplementary Methods for additional details. Phylogenetic analysis A species-level phylogenetic analysis was conducted based on a new data matrix comprising 16 in-group taxa and 50 morphological characters that incorporate the new comparative morphometric data (see Supplementary Methods , Supplementary Note S2 and Supplementary Table S4 ). Parsimony was used as the selection criterion under standard parameters, and both bootstrap and Bremer decay support values were calculated (details in Supplementary Methods ). To time-calibrate the phylogeny, a single tree needed to be selected. To choose between the resulting most parsimonious trees, we used the Stratigraphic Consistency Index and the Gap Excess Ratio based on the age of each taxon. These methods were consistent in their results and allowed us to select the single most stratigraphically consistent MPT to use for time calibration of the phylogeny ( Fig. 5 ). Time calibration was carried out to the highest resolution possible for each taxon using published data [23] , [24] , [25] corrected based on our data as necessary. Species richness, for both observed and ghost taxa, was calculated at the substage level. Pachycephalosaur taphonomy Taphonomic data on virtually all known pachycephalosaur specimens (excluding isolated teeth) were collected based on knowledge of museum collections. This data set consists of 575 specimens from the Cretaceous of North America and Asia. For each specimen, the housing institution, genus, geological formation of origin, and if the material consisted of isolated cranial, isolated postcranial or an articulated/associated specimen was recorded ( Supplementary Table S5 ). Ornithischian diversity Records of ornithischian diversity through the final three stages of the Late Cretaceous were obtained from the Paleobiology Database ( www/paleodb.org ). Records for Hadrosauridae, Leptoceratopsidae and Ceratopsidae were obtained using the Count Taxa feature of the PDBD, accessed on 11 August 2012. The Leptoceratopsidae record was corrected using the data in Ryan et al. [47] . Thescelosauridae data was obtained by using the Taxon Counts feature for the constituent North American genera of this family following Brown et al. [46] . Pachycephalosaur data were obtained using the specimen level pachycephalosaur data set ( Supplementary Table S6 ) segregated into total diversity and diversity of taxa known from articulates/associated skeletons. In all cases, occurrence-based species diversity in each time bin was recorded. Nomenclatural act This published work and the nomenclatural acts it contains have been registered in ZooBank, the proposed online registration system for the International Code of Zoological Nomenclature. The ZooBank LSIDs (Life Science Identifiers) can be resolved and the associated information viewed through any standard web browser by appending the LSID to the prefix ‘ http://zoobank.org/ ’. The LSIDs for this publication are: urn:lsid:zoobank.org:act:D9254894-8009-487F-8490-F3090044EC9C; urn:lsid:zoobank.org:pub:CBE485DA-ABDA-42AC-9834-FB6EE9548C3B. In addition, high-resolution CT scans of the holotype specimen were performed by the University of Texas High-Resolution X-ray CT Facility, and visualizations of those scans were provided by the Digital Morphology (DigiMorph) project. The scan data and visualizations can be freely accessed online ( http://digimorph.org/specimens/Acrotholus_audeti/ ). How to cite this article: Evans D. C. et al. The oldest North American pachycephalosaurid and the hidden diversity of small-bodied ornithischian dinosaurs. Nat. Commun. 4:1828 doi:10.1038/ncomms2749 (2013).